Melanoma whole-exome sequencing identifiesV600EB-RAFamplification-mediated acquired B-RAF inhibitor resistance The development of acquired drug resistance hampers the long-term success of B-RAF inhibitor therapy for melanoma patients. Here we show V600E B-RAF copy-number gain as a mechanism of acquired B-RAF inhibitor resistance in 4 out of 20 (20%) patients treated with B-RAF inhibitor. In cell lines, V600E B-RAF overexpression and knockdown conferred B-RAF inhibitor resistance and sensitivity, respectively. In V600E B-RAF amplification-driven (versus mutant N-RAS -driven) B-RAF inhibitor resistance, extracellular signal-regulated kinase reactivation is saturable, with higher doses of vemurafenib down-regulating phosho-extracellular signal-regulated kinase and re-sensitizing melanoma cells to B-RAF inhibitor. These two mechanisms of extracellular signal-regulated kinase reactivation are sensitive to the MEK1/2 inhibitor AZD6244/selumetinib or its combination with the B-RAF inhibitor vemurafenib. In contrast to mutant N-RAS-mediated V600E B-RAF bypass, which is sensitive to C-RAF knockdown, V600E B-RAF amplification-mediated resistance functions largely independently of C-RAF. Thus, alternative clinical strategies may potentially overcome distinct modes of extracellular signal-regulated kinase reactivation underlying acquired B-RAF inhibitor resistance in melanoma. Activating B-RAF V600 kinase mutations occur in ~50% of melanomas [1] , and the ATP-competitive type I RAF inhibitors, PLX4032/vemurafenib and GSK2118436, display remarkable anti-tumour activity leading to overall survival advantage in patients with V600 B-RAF mutant melanomas [2] , [3] , [4] , [5] , [6] . Acquisition of drug resistance leading to clinical relapse, however, develops in virtually all patients treated with B-RAF inhibitors (B-RAFi) [4] , [5] . Heterogeneous mechanisms of acquired B-RAFi resistance hitherto uncovered fall into general mitogen-activated protein kinase (MAPK)-redundant, AKT-dependent [7] , [8] or MAPK-reactivating [9] , [10] pathways, indicating specific translatable therapeutic strategies to prevent or overcome resistance. Contrary to expectation, V600E B-RAF secondary mutations have not been found to account for acquired B-RAFi resistance [10] , suggesting V600E B-RAF-bypass mechanisms as the principal means to extracellular signal-regulated kinase (ERK) reactivation. Here we observed an alteration in V600E B-RAF , namely genomic copy-number gain, in tumours of melanoma patients whose cancer progressed after initial responses to B-RAFis. We demonstrated that this V600E B-RAF amplification results in V600E B-RAF overexpression, which is necessary and sufficient for acquired resistance to B-RAFi. This finding, along with a recent study reporting amino-terminal truncation of V600E B-RAF causing acquired B-RAFi resistance in melanoma [11] , underscores key molecular alterations in the drug target itself. We further suggest that V600E B-RAF-instrinsic (overexpression, truncation) versus V600E B-RAF-bypass (N-RAS mutations) mechanisms, both reactivating the MAPK pathway, may offer insights into distinct therapeutic strategies to overcome acquired B-RAFi resistance in melanoma. Whole-exome sequencing identifies V600E B-RAF amplification. We assembled 20 sets of patient-matched baseline (before B-RAFi therapy) and disease progression (DP; that is, acquired B-RAFi resistance) melanoma tissues and analysed them to identify the proposed mechanisms of acquired B-RAFi resistance in melanoma. These reported mechanisms include N-RAS [10] and MEK1 (ref. 12 ) mutations, alternative-spliced V600E B-RAF variants [11] , and overexpression of receptor tyrosine kinases (RTKs) (PDGFRβ [7] , [10] , IGF1-R [8] ) and COT [9] ( Tables 1 and Supplementary Table S1 and Fig. S1 ). For DP samples negative for these mechanisms and where there was sufficient frozen and patient-matched normal tissues (from patients no. 4, 5, 8, 14, 16, 17 and 18), we subjected triads of genomic DNAs (gDNAs) from normal, baseline and DP tissues to whole-exome sequencing. In two available data sets, we searched for somatic DP-specific non-synonymous single-nucleotide variants (snSNVs) and small insertion-deletion (indels), which were exceedingly few in number or absent, respectively, using our bioinformatic workflow ( Supplementary Tables S2 and S3 ). We also analysed for DP-specific copy-number variations (CNVs) from the exome sequence data ( Supplementary Table S2 ). This identified V600E B-RAF copy-number gains in these two patients' DP tissues (2.2- and 12.8-fold in patients no. 5 and 8, respectively) relative to their respective baseline tissues ( Fig. 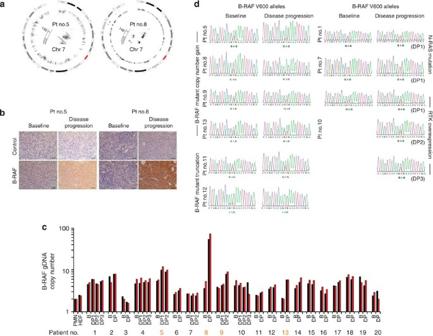Figure 1: Exome sequencing identifiesV600EB-RAFamplification as a candidate mechanism for BRAFi resistance. (a) Copy-number variations (CNVs) called from whole-exome sequence data on two triads of gDNAs using ExomeCNV and chromosome 7 as visualized by Circos (outer ring, genomic coordinates (Mbp); centromere, red; inner ring, log ratio values between baseline and disease progression (DP) samples' average read depth per each capture interval; scale of axis for patient no. 5 –5 to 5 and for patient no. 8 –2.5 to 2.5). Two patients whose melanoma responded to and then progressed on vemurafenib. The genomic region coded orange (magnified views shown in the center of Circos maps) represents the location of B-RAF (chr7:140,424,943-140,524,564), which shows an average log ratio value of 1.14 (2.2-fold gain; patient no. 5) and 3.8 (12.8-fold gain; patient no. 8). (b) B-RAF immunohistochemistry on paired tissues derived from the corresponding patients as ina(scale bar, 50 μM). (c) Validation ofV600EB-RAFcopy-number gain by gDNA Q–PCR (black and red by B-RAF primer set 1 and 2, respectively) and recurrence across distinct patients (positives highlighted in orange). PMN, peripheral mononuclear cells; HDF, human dermal fibroblasts for diploid gDNAs. (d)B-RAFV600 mutant to WT ratio increases with disease progression or acquisition of B-RAFi resistance mediated by mutantB-RAFcopy-number gain. Chromatograms from Sanger sequencing for melanoma samples from patients who acquired B-RAFi resistance based on distinct molecular alterations:V600EB-RAFcopy-number gain,V600EB-RAFtruncation,N-RASmutation or RTK overexpression. 1a ; Table 1 ). Gain in V600E B-RAF copy number was reflected in corresponding increased gene expression at the protein level ( Fig. 1b ). Table 1 Clinical characteristics and acquired resistance mechanisms in patients with matched baseline and DP melanomas tissues. Full size table Figure 1: Exome sequencing identifies V600E B-RAF amplification as a candidate mechanism for BRAFi resistance. ( a ) Copy-number variations (CNVs) called from whole-exome sequence data on two triads of gDNAs using ExomeCNV and chromosome 7 as visualized by Circos (outer ring, genomic coordinates (Mbp); centromere, red; inner ring, log ratio values between baseline and disease progression (DP) samples' average read depth per each capture interval; scale of axis for patient no. 5 –5 to 5 and for patient no. 8 –2.5 to 2.5). Two patients whose melanoma responded to and then progressed on vemurafenib. The genomic region coded orange (magnified views shown in the center of Circos maps) represents the location of B-RAF (chr7:140,424,943-140,524,564), which shows an average log ratio value of 1.14 (2.2-fold gain; patient no. 5) and 3.8 (12.8-fold gain; patient no. 8). ( b ) B-RAF immunohistochemistry on paired tissues derived from the corresponding patients as in a (scale bar, 50 μM). ( c ) Validation of V600E B-RAF copy-number gain by gDNA Q–PCR (black and red by B-RAF primer set 1 and 2, respectively) and recurrence across distinct patients (positives highlighted in orange). PMN, peripheral mononuclear cells; HDF, human dermal fibroblasts for diploid gDNAs. ( d ) B-RAF V600 mutant to WT ratio increases with disease progression or acquisition of B-RAFi resistance mediated by mutant B-RAF copy-number gain. Chromatograms from Sanger sequencing for melanoma samples from patients who acquired B-RAFi resistance based on distinct molecular alterations: V600E B-RAF copy-number gain, V600E B-RAF truncation, N-RAS mutation or RTK overexpression. Full size image V600E B-RAF amplification was validated by gDNA quantitative PCR (Q–PCR), producing consistent fold increases in DP-specific V600E B-RAF copy-number gain (relative to baseline; 2.0- and 14-fold increase in patient no. 5 and 8, respectively; Fig. 1c ). We then expanded the analysis of V600E B-RAF amplification to all 20 paired melanoma tissues and detected V600E B-RAF copy-number gains in DP samples from two additional patients (2.3- and 3-fold for DP2 of patient no. 9 and DP of patient no. 13, respectively; Fig. 1c ; Table 1 ). We note that these copy-number fold increases are likely underestimates of the true changes due to non-tumour diploid cell contents and tumour heterogeneity, as most disease progressive tumours occur from stable residual tumours as a result of partial responses seen in the vast majority of patients treated with B-RAFis. An increase in the mutant B-RAF to wild-type (WT) B-RAF ratio was also noted in all four cases of DP harbouring B-RAF copy-number gain when compared with their respective baseline tissues ( Fig. 1d ), consistent with selection for V600E B-RAF (versus the WT B-RAF allele) copy-number gain during acquisition of B-RAFi resistance. V600E B-RAF amplification was largely mutually exclusive with N-RAS mutations (no enrichment in MEK1 exon 3 mutation was detected in DP versus baseline tumours), RTK overexpression (no COT overexpression detected), as well as a novel mechanism involving V600E B-RAF alternative splicing [11] ( Table 1 ; Supplementary Fig. S1 ). B-RAFi selects for V600E B-RAF gain and overexpression. We have derived vemurafenib/PLX4032-resistant (R) sublines by providing continuous vemurafenib exposure to seven human melanoma-derived V600E B-RAF -positive parental (P) cell lines sensitive to vemurafenib-mediated growth inhibition. Four resistant sublines, including M229 R5 and M238 R1 (refs 7 , 10 ), overexpressed PDGFRβ compared with their parental counterpart. One subline (M249 R4 (ref. 10 )) gained a mutation in N-RAS , and another (M397 R) an alternatively spliced variant of V600E B-RAF resulting in in-frame fusion of exons 1 and 11 ( Supplementary Fig. S2 ). As in our tissue analysis, these mechanisms were identified in a mutually exclusive manner. Another vemurafenib-resistant subline, M395 R, was derived from a V600E B-RAF -homozygous parental line, M395 P ( Supplementary Fig. S3a ). Compared with M395 P, M395 R harbours increased copy numbers of V600E B-RAF gDNA and complementary DNA, consistent with a marked V600E B-RAF protein overexpression ( Supplementary Fig. S3b,c,d ). M395 R displays growth highly resistant to vemurafenib treatment ( Supplementary Fig. S4a ), and titration of M395 R with vemurafenib (1 h) after a 24 h of drug withdrawal revealed phospho-ERK levels to be highly resistant to acute V600E B-RAF inhibition ( Supplementary Fig. S4b ). This pattern of MAPK reactivation was similar to that seen in a mutant N-RAS-driven, vemurafenib-resistant subline, M249 R4, and contrasted with that in the RTK-driven vemurafenib-resistant subline, M229 R5 ( Supplementary Fig. S4b ) [7] , [10] . Expectedly, the levels of p-AKT are unchanged ( Fig. 2b ) comparing M395 P versus M395 R, consistent with a lack of RTK overexpression leading to MAPK-redundant, PI3K-AKT signalling [7] . Accordingly, M395 R does not overexpress either PDGFRβ or IGF-1R, in contrast to M229 R5, which has been shown to overexpress the RTK PDGFRβ ( Supplementary Fig. S4c ) [7] , [8] . In addition, M395 R is WT for N-, H- and K-RAS and MEK1, harbours no secondary mutations in V600E B-RAF or an alternatively spliced variant of V600E B-RAF , which results in a N-terminally truncated V600E B-RAF protein. 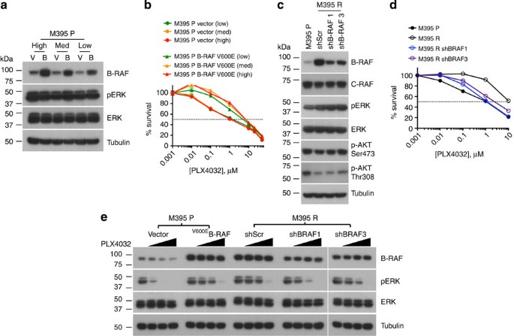Figure 2:V600EB-RAF levels modulate melanoma sensitivity to vemurafenib. (a,b) Western blot showing thatV600EB-RAF overexpression at levels shown did not alter the phospho-ERK (pERK) level in the absence of vemurafenib/PLX4032 (tubulin as loading control) but conferred growth resistance to the parental line, M395 P, when exposed to indicated concentrations of PLX4032 for 72 h (relative to DMSO-treated controls; mean±s.e.m.,n=5). Dashed line, 50% inhibition. (c,d) Transduction of shRNA to knockdown BRAFV600Ein the drug-resistant subline, M395 R, did not alter the pERK level in the absence of PLX4032 but restored growth sensitivity to PLX4032 (72 h; mean±s.e.m.,n=5). (e) Increasing (in M395 P) or decreasing (in M395 R) BRAFV600Elevels decreased or increased pERK sensitivity to PLX4032 (0, 0.1, 1, 10 μM) treatments for 1 h, respectively. Figure 2: V600E B-RAF levels modulate melanoma sensitivity to vemurafenib. ( a , b ) Western blot showing that V600E B-RAF overexpression at levels shown did not alter the phospho-ERK (pERK) level in the absence of vemurafenib/PLX4032 (tubulin as loading control) but conferred growth resistance to the parental line, M395 P, when exposed to indicated concentrations of PLX4032 for 72 h (relative to DMSO-treated controls; mean±s.e.m., n =5). Dashed line, 50% inhibition. ( c , d ) Transduction of shRNA to knockdown BRAF V600E in the drug-resistant subline, M395 R, did not alter the pERK level in the absence of PLX4032 but restored growth sensitivity to PLX4032 (72 h; mean±s.e.m., n =5). ( e ) Increasing (in M395 P) or decreasing (in M395 R) BRAF V600E levels decreased or increased pERK sensitivity to PLX4032 (0, 0.1, 1, 10 μM) treatments for 1 h, respectively. Full size image V600E B-RAF overexpression correlates with B-RAFi resistance. Three different but uniformly modest levels of V600E B-RAF overexpression were achieved by infecting M395 P with varying viral titres and subsequent puromycin selection. This resulted in relatively low (1.9-fold over empty vector virus control), medium (2.4-fold) and high (2.8-fold) levels of V600E B-RAF RNA/cDNA overexpression ( Supplementary Fig. S5 ), with the corresponding protein overexpression levels shown in Fig. 2a . In comparison, in two sets of tissues (from patients no. 8 and 13), where flash-frozen tissues were available, the RNA/cDNA levels of V600E B-RAF in the DP tumours were 9.5- and 1.4-fold relative to those in their patient-matched baseline tumours. Notably, the DP tumour from patient no.13 was obtained by an intervention radiology-guided needle biopsy of a pelvic mass ( Supplementary Table S1 ) and contained a high admixture of normal and tumour contents (latter indicated by S100), which likely contributed to an underestimation of the true change in the V600E B-RAF RNA/cDNA levels. V600E B-RAF overexpression leads to drug-saturable resistance. The modest and incremental overexpression of V600E B-RAF at the RNA and protein levels in M395 P conferred similar degrees of vemurafenib resistance ( Fig. 2b ). Interestingly, further V600E B-RAF overexpression at a much greater level, as in the case of M395 R relative to M395 P (increase in RNA/cDNA level shown in Supplementary Figs S3c and S5 ; increase in protein level shown in Fig. 2c ) conferred enhanced drug resistance mainly at 1 μM vemurafenib but not 10 μM vemurafenib ( Fig. 2d ). Thus, a modest V600E B-RAF copy-number gain and overexpression can confer vemurafenib resistance, and even high amplitude V600E B-RAF amplification and overexpression can be readily saturable by micromolar concentrations of vemurafenib. Moreover, V600E B-RAF knockdown in M395 R confers vemurafenib sensitivity ( Fig. 2c and d ). Consistently, V600E B-RAF overexpression in M395 P (at a level titrated to be comparable to M395 R) and its knockdown in M395 R resulted in pERK resistance and sensitivity, respectively, to acute vemurafenib treatment after a 24 h drug withdrawal ( Fig. 2e ). We predicted that, regardless of the cellular genetic context, MAPK reactivation due to drug target (that is, V600E B-RAF) overexpression would be saturable by higher doses of vemurafenib, in contrast to mutant N-RAS-mediated MAPK reactivation where V600E B-RAF may be bypassed by the alternative use of C-RAF [13] . Indeed, dosing of vemurafenib from 1 to 50 μM revealed a significant difference in drug sensitivity of M249 R4 ( Q61K N-RAS ) versus M395 R (amplified V600E B-RAF ; Fig. 3a; where the latter was highly sensitive to vemurafenib at this drug concentration range), suggesting a potential therapeutic opportunity. To rule out that these results were not due to a difference in genetic backgrounds, we artificially rendered the V600E B-RAF melanoma cell line, M229, vemurafenib-resistant by either Q61K N-RAS or V600E B-RAF viral transduction ( Fig. 3b ). Again, high dose vemurafenib treatment was more effective at overcoming drug resistance in V600E B-RAF-transduced M229 than in the same cell line transduced with Q61K N-RAS. 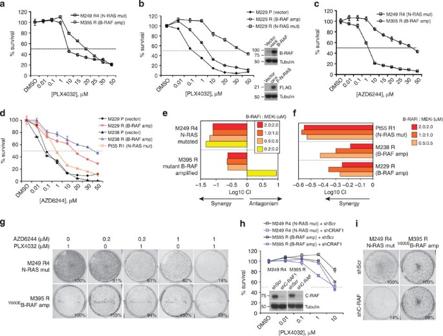Figure 3: Differential B-RAFi/MEKi sensitivities and C-RAF dependency. (a) Survival curves of B-RAFi-acquired resistant sublines, with indicated mechanisms of resistance, to 72 h of B-RAFi (PLX4032) treatments, showcasing differential responses at the micromolar drug range. Results are shown relative to DMSO-treated controls (mean±s.e.m.,n=5; dashed line, 50% inhibition). (b) Survival curves of cell lines, engineered by viral transduction of M229 P to be B-RAFi resistant, to 72 h of B-RAFi (PLX4032) treatments, showcasing differential responses at the micromolar drug range. Results are shown relative to DMSO-treated controls (mean±s.e.m.,n=5). Expression of indicated viral expression constructs shown in western blots. (c) Survival curves of B-RAFi-acquired resistant sublines, with indicated mechanisms of resistance, to 72 h of MEKi (AZD6244) treatments, showcasing differential responses at the micromolar drug range. Results are shown relative to DMSO-treated controls (mean±s.e.m.,n=5). (d) Survival curves of cell lines (engineered by viral transduction of M229 P and M238 P to overexpressV600EB-RAF rendering these parental cells resistant to B-RAFi) to 72 h of MEKi (AZD6244) treatments, showcasing differential responses at the micromolar drug range. Pt55 R (doubleB-RAFandN-RASmutant) is a short-term melanoma culture derived from a tumour, which acquired PLX4032 (vemurafenib) resistance in a treated patient. Results are shown relative to DMSO-treated controls (mean±s.e.m.,n=5). (e,f) Indicated cell lines were treated with constant ratios of PLX4032 and AZD6244 and survival measured after 72 h. Relative synergies, expressed as log10of CI values, are shown. (g) M249 R4 and M395 R were seeded at single-cell density and treated with indicated concentrations of PLX4032 and/or AZD6244. Inhibitors and media were replenished every 2 days, colonies visualized by crystal violet staining after 8 days of drug treatments, and quantified (% growth relative to cells treated with 1 μM PLX4032). Photographs representative of two independent experiments. (h) Survival curves of indicated cell lines after shScrambled or shC-RAF transduction (inset) and when treated with PLX4032 for 72 h. (i) Clonogenic assays of cell lines inewith 14 days (M249 R4) or 18 days (M395 R) of PLX4032 treatment. Results are representative of two experiments. Figure 3: Differential B-RAFi/MEKi sensitivities and C-RAF dependency. ( a ) Survival curves of B-RAFi-acquired resistant sublines, with indicated mechanisms of resistance, to 72 h of B-RAFi (PLX4032) treatments, showcasing differential responses at the micromolar drug range. Results are shown relative to DMSO-treated controls (mean±s.e.m., n =5; dashed line, 50% inhibition). ( b ) Survival curves of cell lines, engineered by viral transduction of M229 P to be B-RAFi resistant, to 72 h of B-RAFi (PLX4032) treatments, showcasing differential responses at the micromolar drug range. Results are shown relative to DMSO-treated controls (mean±s.e.m., n =5). Expression of indicated viral expression constructs shown in western blots. ( c ) Survival curves of B-RAFi-acquired resistant sublines, with indicated mechanisms of resistance, to 72 h of MEKi (AZD6244) treatments, showcasing differential responses at the micromolar drug range. Results are shown relative to DMSO-treated controls (mean±s.e.m., n =5). ( d ) Survival curves of cell lines (engineered by viral transduction of M229 P and M238 P to overexpress V600E B-RAF rendering these parental cells resistant to B-RAFi) to 72 h of MEKi (AZD6244) treatments, showcasing differential responses at the micromolar drug range. Pt55 R (double B-RAF and N-RAS mutant) is a short-term melanoma culture derived from a tumour, which acquired PLX4032 (vemurafenib) resistance in a treated patient. Results are shown relative to DMSO-treated controls (mean±s.e.m., n =5). ( e , f ) Indicated cell lines were treated with constant ratios of PLX4032 and AZD6244 and survival measured after 72 h. Relative synergies, expressed as log 10 of CI values, are shown. ( g ) M249 R4 and M395 R were seeded at single-cell density and treated with indicated concentrations of PLX4032 and/or AZD6244. Inhibitors and media were replenished every 2 days, colonies visualized by crystal violet staining after 8 days of drug treatments, and quantified (% growth relative to cells treated with 1 μM PLX4032). Photographs representative of two independent experiments. ( h ) Survival curves of indicated cell lines after shScrambled or shC-RAF transduction (inset) and when treated with PLX4032 for 72 h. ( i ) Clonogenic assays of cell lines in e with 14 days (M249 R4) or 18 days (M395 R) of PLX4032 treatment. Results are representative of two experiments. Full size image MEK inhibition restores vemurafenib sensitivity. As both N-RAS mutation and V600E B-RAF amplification-driven acquired resistance mechanisms would be anticipated to result in MEK reactivation, we tested the allosteric MEK inhibitor (MEKi), AZD6244/selumetinib, on the Q61K N-RAS -driven M249 R4 and the V600E B-RAF amplification-driven M395 R sublines. MEKi treatment resulted in decreased proliferation in both cases, but the activity was noted at lower concentrations for the Q61K N-RAS -driven resistance mechanism ( Fig. 3c ). This differential pattern was reproducible by exposing AZD6244/selumetinib to V600E B-RAF melanoma cell lines M229 and M238 transduced with high levels of V600E B-RAF versus a short-term culture, Pt55 R [10] , with Q61K N-RAS -driven acquired B-RAFi resistance ( Fig. 3d ). We also tested the combination of B-RAFi with MEKi, which is currently in clinical testing [14] , in 3-day survival assays. A calculation of combination index (CI) values using equal ratios of vemurafenib and selumetinib was performed. The results were consistent with a highly synergistic effect of these two agents combined in overcoming both mutant N-RAS -driven (M249 R4) and V600E B-RAF amplification-driven B-RAFi resistance (M395 R; Fig 3e,f ), although the combination tended to be more potent against mutant N-RAS-driven acquired resistance to vemurafenib. This B-RAFi and MEKi combinatorial synergy was further corroborated in longer-term clonogenic assays ( Fig. 3g ). Differential C-RAF dependency of ERK-reactivating mechanisms. We also predicted that MAPK reactivation due to V600E B-RAF overexpression would be C-RAF-independent, in contrast to mutant N-RAS-mediated MAPK reactivation where V600E B-RAF may be bypassed by the alternative use of C-RAF. Indeed, C-RAF knockdown by short hairpin RNA (shRNA) sensitized the mutant N-RAS subline, M249 R4, but not the V600E B-RAF amplified subline, M395 R, to vemurafenib in 3-day survival assays ( Fig. 3h ). C-RAF knockdown restored vemurafenib sensitivity to M249 R4 ( Q61K N-RAS / V600E B-RAF ) even more strikingly in a longer-term clonogenic assays, which afforded fresh drug replacement every 2 days ( Fig. 3i ). An independent C-RAF shRNA also restored vemurafenib sensitivity to M249 R4 ( Supplementary Table S4 ). In addition, B-RAFi and MEKi synergy and C-RAF-dependence in mutant N-RAS-driven acquired B-RAFi resistance was confirmed in a short-term culture derived from a tumour with clinical acquired vemurafenib resistance ( Supplementary Fig. S6 ). Identification of V600E B-RAF amplification as a mechanism of acquired resistance in B-RAFi-treated patients provides evidence for alterations in the drug target causing clinical relapse. Based on these studies, therapeutic stratification of MAPK reactivation underlying B-RAFi resistance into drug-saturable or C-RAF-dependent pathways may be translatable into the design of next-generation clinical trials aimed at preventing or overcoming B-RAFi resistance ( Fig. 4 ). These findings also provide pre-clinical rationale for dose escalation studies in selected patients with B-RAFi-resistant V600E/K B-RAF metastatic melanomas, particularly given the wide range of effective dosing and the fact that the maximum tolerated dose of GSK2118436 has not been determined. The combination of current B-RAFis (or next-generation RAF inhibitors that enhance B-RAF potency or feature pan-RAF inhibition) with MEK1/2 inhibitors may potentially broadly block MAPK reactivation. 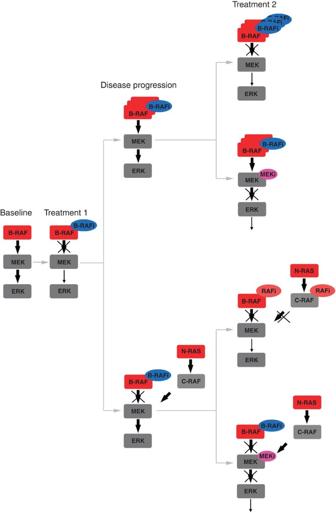Figure 4: MAPK-reactivating mechanisms of acquired B-RAFi resistance and therapeutic implications. Distinct strategies to overcome acquired resistance driven by amplification of mutantB-RAFor mutations inN-RAS. Schematic of ERK-reactivating pathways (V600EB-RAFamplification indicated by stacked symbols, top;N-RASmutation, bottom; mutant proteins in red and WT proteins in grey) and proposed strategies to restore B-RAFi sensitivity (increasing B-RAFi concentration or potency, top; switching B-RAFi to pan-RAFi, bottom). Alternatively, the combination of B-RAFi and MEKi are predicted to synergistically growth-inhibit melanomas with acquired resistance to B-RAFi monotherapy stemming from ERK reactivation. Figure 4: MAPK-reactivating mechanisms of acquired B-RAFi resistance and therapeutic implications. Distinct strategies to overcome acquired resistance driven by amplification of mutant B-RAF or mutations in N-RAS . Schematic of ERK-reactivating pathways ( V600E B-RAF amplification indicated by stacked symbols, top; N-RAS mutation, bottom; mutant proteins in red and WT proteins in grey) and proposed strategies to restore B-RAFi sensitivity (increasing B-RAFi concentration or potency, top; switching B-RAFi to pan-RAFi, bottom). Alternatively, the combination of B-RAFi and MEKi are predicted to synergistically growth-inhibit melanomas with acquired resistance to B-RAFi monotherapy stemming from ERK reactivation. Full size image Emerging evidence points to B-RAF mutant cancers of other tissue origin or lineage being less responsive to specific B-RAF inhibition than B-RAF mutant melanomas. Mechanisms of acquired B-RAFi resistance may turn out to be instructive for understanding primary resistance of B-RAF mutant cancer types to B-RAFis, as primary (de novo) and secondary (or acquired) drug resistance may be clinical manifestations from a spectrum of molecular alterations that are mechanistically linked. Thus, multiple modes (for example, mutation, copy-number gain) of up-regulating oncogene activity, which may pre-exist in the same tumour and/or patient, may help to explain the range of heterogeneous responses of B-RAF mutant cancers to direct B-RAF, MEK or ERK inhibition. Cell culture experiments Cells were maintained in DMEM with 10 or 20% fetal bovine serum and glutamine. shRNAs ( Supplementary Table S4 ) for B-RAF and C-RAF were subcloned into the lentiviral vector pLL3.7; pBabe B-RAF (V600E) was purchased from (plasmid 17544) Addgene; viral supernatants generated by co-transfection with three packaging plasmids into HEK293T cells; and infections carried out with protamine sulphate. Stocks and dilutions of PLX4032 (Plexxikon, Berkeley, CA, USA) and AZD6244 (commercially available) were made in DMSO. Cells were quantified using CellTiter-GLO Luminescence (Promega) or crystal violet staining followed by NIH Image J quantification. Whole-exome sequencing Human tissues were obtained with patient-informed consent under UCLA Institutional Review Board (no. 10-001089) approval. For each sample, 3 μg of high-molecular-weight gDNA was used as the starting material to generate the sequencing library. Exome captures were performed using Agilent SureSelect Human All Exon 50 mb and Agilent SureSelect Human All Exon 50 mb XT for patient no. 5 and 8, respectively, per manufacturers' recommendation, to create a mean 200 bp insert library. For patient no. 5, sequencing was performed on Illumina GenomeAnalyzerII (GAII) as 76+76 bp paired-end run. The normal sample was run on one flowcell lane and the tumour samples were run on two flowcell lanes each. For patient no. 8, sequencing was performed on Illumina HiSeq2000 as 50+50 bp paired-end run and 100+100 bp paired-end run. The three samples (normal, baseline and DP) were initially mixed with nine other samples and run across five flowcell lanes for the 50+50 bp run. For the 100+100 bp run, they were mixed with three other samples to be run across five flowcell lanes with barcoding of each individual genomic sample library. For patient no. 5, approximately 62 million, 137 million and 147 million reads were generated for normal tissue (skin), baseline melanoma and DP melanoma, respectively, with 75.2%, 78.1% and 74.7% of the reads mapping to capture targets. Based on an analysis of reads that uniquely aligned to the reference genome and for which the potential PCR duplicates were removed, an average coverage of 52X, 88X and 114X was achieved with 87%, 92% and 93% of the targeted bases being covered at 10X or greater read depth for normal, baseline and DP, respectively. For patient no. 8, approximately 198 million, 270 million and 256 million reads were generated for normal tissue (skin), baseline melanoma and DP melanoma, respectively, with 43.2%, 44.1% and 42.3% of the reads mapping to capture targets. Based on an analysis of reads that uniquely aligned to the reference genome and for which the potential PCR duplicates were removed, an average read depth of 107X, 132X and 123X was achieved with 89%, 90% and 90% of the targeted bases being covered at 10X or greater for normal, baseline and DP, respectively. Sequencing data analysis. For patient no. 8 where the samples were indexed and pooled before the sequencing, Novobarcode from Novocraft was used to de-multiplex the data. The sequence reads were aligned to the human reference genome using Novoalign V2.07.13 from Novocraft ( http://www.novocraft.com ). For patient no. 5, hg18 downloaded from UCSC genome database was used and for patient no.8, b37 downloaded from GATK (Genome analysis toolkit; http://www.broadinstitute.org/gsa/wiki/index.php/GATK_resource_bundle#b37_resources:_the_standard_data_set ) resources website was used for the reference genome. SAMtools v.0.1.16 (ref. 16 ) was used to sort and merge the data and Picard ( http://picard.sourceforge.net/ ) was used to mark PCR duplicates. To correct the misalignments due to the presence of indels, local realignment was performed using RealignerTargetCreator and IndelRealigner of GATK [17] . Indel calls in dbSNP132 were used as known indel input. Then, GATK CountCovariates and TableRecalibration were used to recalibrate the originally reported quality score by using the position of the nucleotide within the read and the preceding and current nucleotide information. Finally, to call the single-nucleotide variants (SNVs), the GATK UnifiedGenotyper was used to the realigned and re-calibrated bam file while GATK IndelGenotyperV2 was used to call small insertion/deletions (Indels). To generate a list of somatic variants for DP tumour, the difference in allele distribution was calculated using one-sided Fisher's exact test using normal sample or the baseline sample. Variants with P -value <0.05 were included in the 'somatic variant list'. Low coverage (<10X) SNVs and SNVs with more than one variant allele in normal tissue and baseline melanoma were filtered out during the process. These somatic variants were further annotated with SeattleSeqSNPannotation ( http://gvs.gs.washington.edu/SeattleSeqAnnotation/ ). For DP-specific, non-synonymous SNVs that result in missense mutations, we assessed the level of amino-acid conservation using PhyloP score (provided in UCSC genome database) where a score >2 implies high conservation and the nature of amino substitution using Polyphen-2 analysis [18] . CNV analysis was performed using an R package, ExomeCNV [15] . ExomeCNV uses the ratio of read depth between two samples at each capture interval. Here, the read depth data between baseline and DP melanomas were compared. Briefly, the read depth information was extracted through the PILEUP file generated from the BAM file after removing PCR duplicates using SAMtools. The average read depth at each capture interval was calculated and the classify.eCNV module of ExomeCNV was run with the default parameters to calculate the copy-number estimate for each interval. Subsequently, another R package commonly used to segment the copy-number intervals, DNAcopy [19] , was called through ExomeCNV multi.CNV.analyze module with default parameters to do segmentation and sequential merging. The genomic regions with copy number 1 were called deletion and any regions with copy number >2 were called amplification. Circos [20] was used to visualize the CNV data. Protein detection Western blots were probed with antibodies against p-ERK1/2 (T202/Y204), ERK1/2, C-RAF, AKT (Ser473), AKT (Thr308), AKT (Cell Signaling Technologies; all at 1:1,000), N-RAS, B-RAF (Santa Cruz Biotechnology; both at 1:500) and tubulin (Sigma; 1:700). For B-RAF immunohistochemistry, paraffin-embedded formalin-fixed tissue sections were antigen-retrieved, incubated with the primary antibody (Santa Cruz Biotechnology; 1:50) followed by HRP-conjugated secondary antibody (Envision System, DakoCytomation). Immunocomplexes were visualized using the DAB (3,3′-diaminobenzidine) peroxidase method and nuclei were counterstained with hematoxylin. Genomic DNA and RNA quantifications For real-time Q–PCR, total RNA was extracted and cDNA quantified by the iCycler iQ Real-Time PCR Detection System (Bio-Rad). Data were normalized to TUBULIN and GAPDH levels. Relative expression is calculated using the delta-Ct method. gDNAs were extracted using the FlexiGene DNA Kit (Qiagen; Human Genomic DNA-Female, Promega). B-RAF relative copy number was determined by Q–PCR (cycle conditions available upon request) using the MyiQ single colour Real-Time PCR Detection System. Total DNA content was estimated by assaying β-globin for each sample, and 20 ng of gDNA was mixed with the SYBR Green Q–PCR Master Mix (Bio-Rad) and 2 pmol l −1 of each primer. All primer sequences are provided in Supplementary Table S4 . Data processing Statistical analyses were performed using InStat 3 Version 3.0b (GraphPad Software); graphical representations using DeltaGraph or Prism (Red Rock Software); and CI calculation using CalcuSyn V2.1 (Biosoft). Calculations were made by CalcuSyn software using the method of Chou and Taladay. Interpretation of CI values is summarized as follows: CI <0.1 (very strong synergy); 0.1–0.3 (strong synergy); 0.3–0.7 (synergy); 0.7–0.85 (moderate synergy); 0.85–0.9 (slight synergy); 0.90–1.10 (nearly additive); and 1.10–1.20 (slight antagonism). The relevant correlated Log 10 (CI) values are shown as follow: Log 10 (CI 0.1)=−1; Log 10 (CI 0.3)=−0.5228787452803376; Log 10 (CI 0.7)=−0.1549019599857432 and Log 10 (CI 0.85)=−0.07058107428570727. Accession codes: Sequence data are archived at the NCBI Sequence Read Archive (SRA) under the accession code SRP010266 . How to cite this article: Shi, H. et al . Melanoma whole-exome sequencing identifies V600E B-RAF amplification-mediated acquired B-RAF inhibitor resistance. Nat. Commun. 3:724 doi: 10.1038/ncomms1727 (2012).